Superconductivity-induced optical anomaly in an iron arsenide One of the central tenets of conventional theories of superconductivity, including most models proposed for the recently discovered iron-pnictide superconductors, is the notion that only electronic excitations with energies comparable to the superconducting energy gap are affected by the transition. Here, we report the results of a comprehensive spectroscopic ellipsometry study of a high-quality crystal of superconducting Ba 0.68 K 0.32 Fe 2 As 2 that challenges this notion. We observe a superconductivity-induced suppression of an absorption band at an energy of 2.5 eV, two orders of magnitude above the superconducting gap energy 2Δ≈20 meV. On the basis of density functional calculations, this band can be assigned to transitions from As-p to Fe-d orbitals crossing the Fermi level. We identify a related effect at the spin-density wave transition in parent compounds of the 122 family. This suggests that As-p states deep below the Fermi level contribute to the formation of the superconducting and spin-density wave states in the iron arsenides. The standard Bardeen–Cooper–Schrieffer (BCS) theory of superconductivity, based solely on an effective attractive interaction between electrons mediated by phonons, does not provide a satisfactory explanation of the properties of strongly correlated high-temperature superconductors. Theoretical proposals in earlier years suggest that electronic excitations might enhance this interaction and thus contribute to the formation of the superconducting condensate [1] , [2] , [3] , [4] , [5] . These proposals appeared to gain some ground with the observation of superconductivity-induced transfer of the optical spectral weight (SW) in the cuprate high-temperature superconductors, which involves a high-energy scale extending to the visible range of the spectrum [6] . In spite of numerous studies (for a comprehensive list of references see ref. 7 ), no modification of interband optical transitions in the superconducting state has been directly identified in the cuprates. Instead, the observed superconductivity-induced anomalies in the optical response of highly conducting CuO 2 planes were found to be confined to the energy range corresponding to transitions within the conduction band below the plasma edge. These changes are dominated by the narrowing of the broad Drude peak caused by a superconductivity-induced modification of the scattering rate [8] , [9] , [10] . A minute redistribution of the SW between the conduction band and high-energy Hubbard bands generated by Coulomb correlations may also play a role [11] , [12] . Current research on the recently discovered iron-pnictide superconductors [13] suggests that electronic correlations are weaker than those in the cuprates. Unlike in cuprates, the Fermi surface has been reliably determined over the entire phase diagram and shows good agreement with density functional calculations. The superconducting state of the iron-pnictides appears to fit well into a BCS framework in which phonons, which in these compounds interact only weakly with electrons [14] , are replaced by spin fluctuations [15] . The ellipsometric data we present here are consistent with the hypothesis that electronic correlations result in only a modest renormalization of the electronic states. However, the superconductivity-induced optical anomalies we observed involve modification of an absorption band at an energy of 2.5 eV, two orders of magnitude greater than the superconducting gap 2Δ≈20 meV. In contrast to the cuprate superconductors, this high-energy anomaly has a regular Lorentzian shape in both the real and imaginary parts of the dielectric function and is confined to energies well above the plasma edge ω pl ≈1.6 eV. It can be explained as a consequence of non-conservation of the total number of unoccupied states involved in the corresponding optical transitions due to the opening of the superconducting gap. This implies that unconventional interactions beyond the BCS framework must be considered in models of the superconducting pairing mechanism. Superconductivity-induced optical anomalies in Ba 0.68 K 0.32 Fe 2 As 2 The measurements were carried out on a single crystal of Ba 1− x K x Fe 2 As 2 (BKFA) with x =0.32 and superconducting transition temperature T c =38.5 K. Specific heat measurements on the same sample confirm its high purity and the absence of secondary electronic phases [16] . We performed direct ellipsometric measurements of the in-plane complex dielectric function ɛ ( ω )= ɛ 1 ( ω )+ iɛ 2 ( ω )=1+4π iσ ( ω )/ ω over a range of photon energies extending from the far infrared ( ω 12 meV) to the ultraviolet ( ω 6.5 eV), with subsequent Kramers–Kronig (KK) consistency analysis (see Methods ). The far-infrared optical conductivity is dominated by the opening of a superconducting gap of magnitude 2Δ≈20 meV below T c ( Fig. 1a ), in accordance with previous studies of optimally doped BKFA [17] . The low-energy missing area in the optical conductivity spectrum below T c , is contained within 10Δ and amounts to equivalent to a London penetration depth of λ p 2,200 Å. The fraction of the missing area below 12 meV not accessible to the experiment was accurately quantified from the requirement of KK consistency of the independently measured real and imaginary parts of the dielectric function. 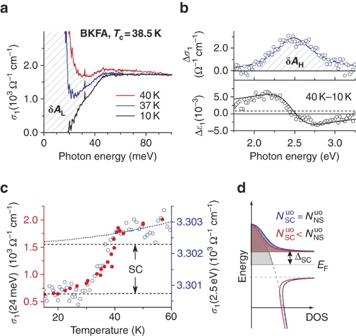Figure 1: Superconductivity-induced anomalies in optical conductivity. (a) Real part of the far-infrared optical conductivity of Ba0.68K0.32Fe2As2and the missing area. (b) Difference spectra of the real part of the optical conductivity (top panel) and dielectric function (bottom panel) between 40 and 10 K, with a small background shift (horizontal dashed line) detected by temperature modulation measurements. Lorentzian fit to both spectra (black solid lines). (c) Temperature scan ofσ1at 2.5 eV. Contribution of the normal-state dynamics (dotted line) was estimated to determine the magnitude of the SC-induced jump (dashed lines). (d) Density of states in the normal (NS; grey dashed line), conventional superconducting state (SC; blue line), and an unconventional state with a depletion of unoccupied states (UO; red line). Filled areas of respective colours represent total number of unoccupied states. Figure 1: Superconductivity-induced anomalies in optical conductivity. ( a ) Real part of the far-infrared optical conductivity of Ba 0.68 K 0.32 Fe 2 As 2 and the missing area. ( b ) Difference spectra of the real part of the optical conductivity (top panel) and dielectric function (bottom panel) between 40 and 10 K, with a small background shift (horizontal dashed line) detected by temperature modulation measurements. Lorentzian fit to both spectra (black solid lines). ( c ) Temperature scan of σ 1 at 2.5 eV. Contribution of the normal-state dynamics (dotted line) was estimated to determine the magnitude of the SC-induced jump (dashed lines). ( d ) Density of states in the normal (NS; grey dashed line), conventional superconducting state (SC; blue line), and an unconventional state with a depletion of unoccupied states (UO; red line). Filled areas of respective colours represent total number of unoccupied states. Full size image Careful examination of the visible range uncovered a superconductivity-induced suppression of an absorption band at 2.5 eV. Figure 1b shows difference spectra between 40 and 10 K of the real parts of the optical conductivity and dielectric function. The suppressed band has a Lorentzian lineshape and appears abruptly across the superconducting transition, consistently in both Δ σ 1 and Δ ɛ 1 , as shown in Figure 1c for σ 1 (2.5 eV). The temperature dependence of the suppression (blue open circles) coincides with that of the far-infrared optical conductivity due to the opening of the superconducting gap (red filled circles). Thus, the onset of superconductivity not only modifies the low-energy quasiparticle response but also affects the overall electronic structure, including interband transitions in the visible range of the spectrum. As the SW loss δA H is not balanced in the vicinity of the absorption band ( Fig. 1b ), our data indicate a SW transfer over a wide energy range. We note that the superconductivity-induced modification of the lattice parameters only results in a minute volume change of Δ V / V ≈5×10 −7 , which is insufficient to explain the optical anomaly (C. Meingast, personal communication). A KK consistency analysis could not be carried out with sufficient accuracy to show whether or not the SW liberated from the absorption band at the superconducting transition contributes to the response of the superconducting condensate at zero energy. We did, however, detect a minute rise in the background level of ɛ 1 (1.5−3.5 eV) below T c , which according to the KK relation implies that the SW is transferred to energies below 1.5 eV. This effect was identified from a simultaneous fit of Δ σ 1 ( ω ) and Δ ɛ 1 ( ω ) (horizontal dashed line in the bottom panel of Fig. 1b ). To estimate the background shift more accurately, temperature modulation measurements of σ 1 at the resonance photon energy 2.47 eV and of ɛ 1 at off-resonance photon energies of 2.12 eV and 2.82 eV were carried out. In Supplementary Figure S1 , the sample temperature was changed between 20 to 40 K with a period of 1,800 s and later averaged over 24 periods to reduce noise to Δ ɛ 1 =10 −4 . This confirms a minute background increase of Δ ɛ 1 (2.47 eV)=(8±4)10 −4 . As the SW δA H liberated from the absorption band upon cooling below T c comprises only ~0.5% of the total SW δA L of the superconducting condensate, its contribution to the low-energy charge dynamics might be considered negligible. However, assuming that this additional high-energy SW contributes to the itinerant-carrier response below T c , a simple estimate in the framework of the tight-binding nearest-neighbour approximation [18] , [19] shows that this would lead to a reduction in electronic kinetic energy of 0.60 meV per unit cell in the superconducting state (see Supplementary Note 1 ). This is close to the condensation energy Δ F (0)=0.36 meV per unit cell obtained from specific heat measurements on the same sample [16] . It is thus important to establish the origin of this unusual optical anomaly. Local density approximation calculations We therefore compared our data with the results of ab initio electronic structure calculations in the framework of the local density approximation (LDA) ( Fig. 2a,b ). A dispersion analysis of the experimental optical conductivity in the range 0.5–6.5 eV yielded three major interband transitions in Ba 0.68 K 0.32 Fe 2 As 2 . A comparison with the LDA results enabled us to identify the initial and final states of these transitions. The lowest-energy transition is located at about 1 eV (red line) and stems from intraband Fe-d and interband As-p to Fe-d transitions. The major contribution to the optical response in the visible spectral range comes from transitions starting from Fe-d or As-p orbitals into strongly hybridized Fe-d to As-p or Fe-d orbitals (green line). Finally, the ultraviolet absorption comes from higher-energy transitions into Ba-d states (blue line). 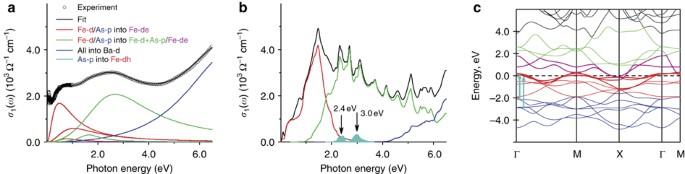Figure 2: Assignment of interband optical transitions. (a) Real part of the optical conductivity of Ba0.68K0.32Fe2As2and contributing interband transitions determined by a dispersion analysis. (b) Corresponding LDA calculation with a breakdown into separate orbital contributions described ina. (c) Band structure from the same LDA calculation. Colour coding of the dispersion curves corresponds to the text colour ina. Superconductivity-suppressed absorption bands (cyan arrows). Figure 2: Assignment of interband optical transitions. ( a ) Real part of the optical conductivity of Ba 0.68 K 0.32 Fe 2 As 2 and contributing interband transitions determined by a dispersion analysis. ( b ) Corresponding LDA calculation with a breakdown into separate orbital contributions described in a . ( c ) Band structure from the same LDA calculation. Colour coding of the dispersion curves corresponds to the text colour in a . Superconductivity-suppressed absorption bands (cyan arrows). Full size image Although the high-energy electronic structure of BKFA is predicted quite well by the LDA calculations, the experimental quasiparticle response due to transitions within the conduction band (or, given the multiorbital structure of iron-pnictides, a narrowly spaced set of conduction bands) shows a significant deviation. The discrepancy can be quantified by the squared ratio of the band-structure plasma frequency (not included in Fig. 2b ) to its experimental counterpart which can be obtained in practice from the residual optical response, after the interband transitions identified using a dispersion analysis have been subtracted. This ratio approximates the quasiparticle effective-mass renormalization factor Such an enhancement is consistent with de Haas-van Alphen and photoemission experiments on other compounds of the 122 family [20] , [21] , [22] and was recently reproduced by combined LDA and dynamical mean-field theory (DMFT) calculations for both 1111 and 122 compounds [23] . These calculations do not show evidence of the formation of Hubbard bands and thus indicate moderate electron–electron correlations. This explains the good agreement of the LDA optical conductivity above 1.5 eV with the experimental data. Now, we turn to the physical origin of the superconductivity-suppressed absorption band. The same LDA calculation revealed a set of interband transitions centered at 2.5 eV, which originate or terminate in states exhibiting hole dispersion and crossing the Fermi level at the Γ- and M-points of the Brillouin zone ( Fig. 2c ). We confidently assign these states to Fe-d yz , zx and Fe-d xy orbitals. The other states involved in these transitions belong to As-p x , y / Fe-d z 2 hybrid orbitals, ~2–3 eV below and above the Fermi level, giving rise to a bandwidth of Δ E ≈1 eV, which is in remarkable agreement with the experiment. Suppression of the absorption band over its full width can be explained by redistribution of the occupation of Fe-d yz , zx and Fe-d xy states under the Fermi level below the superconducting transition. This mechanism is supported by LDA calculations in which the density of states within one superconducting gap energy above the Fermi level was eliminated (see Supplementary Fig. S2 and Method), leading to the observed suppression of the optical transitions shown in cyan in Figure 2b . Spin-density wave-induced SW transfer in SrFe 2 As 2 We have further explored the validity of this scenario by repeating our ellipsometric measurements on parent compounds of the 122 family of iron arsenide superconductors. As the spin-density wave (SDW) instability exhibited by these compounds is also believed to be induced by nesting of electronic states on different electronic bands, we expect an optical anomaly at the SDW transition similar to the one we observed in the superconductor. The magnitude of the anomaly is expected to be greater than the one in the superconductor, because the SDW transition occurs at high temperature and generates a larger energy gap. In SrFe 2 As 2 (SFA), we indeed find a strong reduction in optical absorption upon cooling below T SDW 200 K. The difference spectra of ɛ 1 ( ω ) and ɛ 2 ( ω ) between 200 and 175 K show a double-peak structure, with maxima at 2.4 and 3.4 eV ( Fig. 3a ). A temperature scan across T SDW at the frequency of the second peak (inset of Fig. 3a ) further confirms that this effect is induced by SDW formation. A direct comparison with the superconducting compound is complicated by a pronounced modification of the electronic structure due to the coincident magnetic and structural transitions. 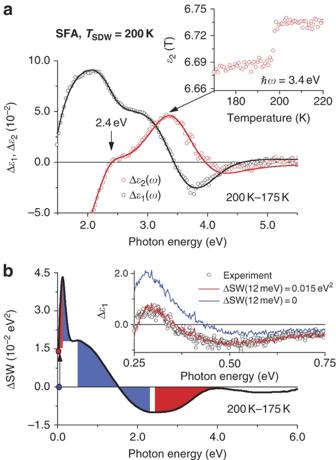Figure 3: SDW-induced anomaly in high-energy optical conductivity. (a) Difference spectra of the real and imaginary parts of the dielectric function of SFA between 200 and 175 K. Lorentzian fit to both (solid lines). (Inset) Temperature scan ofɛ2at 3.4 eV. (b) SW redistribution between 200 and 175 K. SW in the extrapolation region below 12 meV before (blue filled circle) and after (red filled circle) a KK consistency check. Blue and red filled areas represent regions of SW gain and loss, respectively, in the magnetic versus normal state. (Inset) Difference spectra of the real part of the dielectric function obtained experimentally (open circles) and from a KK transformation of the real part of the optical conductivity (solid lines, colours match filled circles). Nevertheless, certain information can be gained from the critical behaviour of the in-plane SW Figure 3b shows difference SW of SFA between 200 and 175 K as a function of the upper integration limit Ω. The change in the SW in the extrapolation region below 12 meV was accurately determined via a KK consistency analysis (see Methods ), as illustrated in the inset of Figure 3b . With ΔSW (12 meV)=0 across the transition (blue filled circle), the KK transformation of the Δ ɛ 2 ( ω ) (blue line) deviates significantly from the experimentally measured Δ ɛ 1 ( ω ). Gradually increasing this SW brings them closer until they finally coincide (red line), thus fixing ΔSW (12 meV)=0.015 eV 2 (red filled circle). The higher-energy redistribution of the SW is broken down in Figure 3b into regions of SW gain (blue areas) and loss (red areas) in the SDW with respect to paramagnetic state. The SW lost because of the opening of the SDW gap [24] (the first red region) is partly transferred to the electronic excitations across the gap (the first blue region) and fully recovered by 1.5 eV. These processes are then followed by high-energy redistribution in the region 1.5–4.0 eV, involving the SW of the suppressed bands. It appears unlikely that such high-energy SW transfer could result from modification of the electronic structure due to a magnetic transition, because effects of electronic reconstruction at the SDW transition are limited by 1.5 eV. A modification of the matrix elements at the structural transitions of sufficient strength cannot account for the observed suppression, because this would be accompanied by an even larger effect at higher energies clearly absent in Figure 3b . A redistribution of charge carriers between the SDW-coupled bands analogous to that in the superconducting compound provides a more natural explanation. The same physical reasons might explain the orbital polarization that breaks the degeneracy of Fe-d xz and Fe-d yz orbitals recently observed in the Ba-based parent of the same family by photoemission spectroscopy [25] . Figure 3: SDW-induced anomaly in high-energy optical conductivity. ( a ) Difference spectra of the real and imaginary parts of the dielectric function of SFA between 200 and 175 K. Lorentzian fit to both (solid lines). (Inset) Temperature scan of ɛ 2 at 3.4 eV. ( b ) SW redistribution between 200 and 175 K. SW in the extrapolation region below 12 meV before (blue filled circle) and after (red filled circle) a KK consistency check. Blue and red filled areas represent regions of SW gain and loss, respectively, in the magnetic versus normal state. (Inset) Difference spectra of the real part of the dielectric function obtained experimentally (open circles) and from a KK transformation of the real part of the optical conductivity (solid lines, colours match filled circles). Full size image The population redistribution required to account for the superconductivity-reduced absorption in BKFA is, however, at variance with the conventional theory of superconductivity. In the framework of the standard BCS approach, opening of an energy gap in a single-band superconductor leads to bending of the quasiparticle dispersion and to expulsion of the density of states in the vicinity of the Fermi surface (grey and blue areas in Fig. 1d ) [26] , with the total number of unoccupied states below the transition conserved (blue area is equal to the grey area in Fig. 1d ). This can only lead to a small corrugation of an optical absorption band on the scale of one superconducting gap energy superimposed on the overall broad feature without any modification of its SW [27] . The experimentally observed suppression of an absorption band on the scale of its full width necessarily requires a population imbalance (red area unequal to the grey area in Fig. 1d ). This effect can be clearly identified as a consequence of superconductivity because the temperature dependence of the suppression mimics that of the optical conductivity in the far-infrared region due to the opening of the superconducting gap, as shown in Figure 1c . All of the iron-pnictide superconductors are known to have multiple superconducting gaps [13] and theoretical work indicates a dominant contribution of electron pairing between different bands to the formation of the superconducting state [15] . Redistribution of the occupation of the different bands below T c could explain the optical anomaly we observed (see Supplementary Fig. S3 ). However, even a generalization of the standard BCS theory to the multiband case [28] does not take this effect into account. It requires lowering the chemical potential of the material in the superconducting state (see Supplementary Note 2 ). In the presence of large Fe-As bond polarizability [29] , [30] , it can potentially enhance superconductivity in iron-pnictides. Interactions of electrons in different energy bands at the Fermi level may provide a common framework for an explanation of the optical anomalies in the SDW and superconducting compounds. It is important to note that these anomalies affect only a small fraction of the interband transitions, which involve initial states of As p -orbital character deep below the Fermi level. This indicates that these orbitals significantly influence electronic instabilities in the iron arsenides, possibly due to the high polarizability of the As–Fe bonds. Our study points to optical SW transfer from high energies to below 1.5 eV induced by collective electronic instabilities. In the superconductor, it occurs at energies two orders of magnitude greater than the superconducting gap energy, suggesting that electronic pairing mechanisms contribute to the formation of the superconducting condensate. Sample preparation The Ba 0.68 K 0.32 Fe 2 As 2 single crystal was grown in zirconia crucibles sealed in quartz ampoules in argon atmosphere [31] . Its chemical composition was determined by energy-dispersive X-ray spectrometry. The quality of the sample and absence of phase separation was confirmed by specific heat experiments that yielded an upper bound of 2.4% (ref. 16 ) on its non-superconducting volume fraction. From direct-current (DC) resistivity, magnetization and specific heat measurement, we obtained T c =38.5±0.2 K. The sample surface was cleaved before every measurement. Experimental apparatus The experimental setup comprises three ellipsometers to cover the spectral range of 12 meV–6.5 eV. For the range 12 meV–1 eV, we used a home-built ellipsometer attached to a standard Fast-Fourier-Transform Bruker 66v/S FTIR interferometer. The far-infrared measurements were performed at the infrared beamline of the Angström Quelle Karlsruhe (ANKA) synchrotron light source at the Karlsruhe Institute of Technology. For the mid-infrared measurements, we used the conventional glow-bar light source from a Bruker 66v/S FTIR. Finally, high-energy spectra 0.7–6.5 eV were measured with a Woollam VASE (variable angle spectroscopic ellipsometer) ellipsometer equipped with an ultra high-vacuum cold-finger cryostat operated at <5×10 −9 mbar chamber pressure. The inherent capacity of Woollam VASE ellipsometers to measure relative changes of the dielectric function in the order of 10 −2 was boosted to an unprecedented level of 10 −4 using temperature-modulation measurements of the dielectric constant at particular photon energies. KK consistency check One of the strong advantages of spectroscopic ellipsometry with respect to reflectometry is that independently obtained real part of the dielectric function Δ ɛ 1 ( ω ) and optical conductivity Δ σ 1 ( ω ) can be used in a KK consistency check, in which Δ ɛ 1 ( ω ) and the KK transform of Δ σ 1 ( ω ) must coincide: This additional constraint unique to ellipsometry allows one to determine with high accuracy the SW in the extrapolation region beyond the experimentally accessible spectral range, in our case below 12 meV. It drastically reduces the extrapolation uncertainty and renders the subsequent data analysis more robust. KK consistency analysis is rather insensitive to the exact shape of the optical spectrum in the extrapolated frequency range, but it does fix the total SW where ω 0 is the experimental low-energy cutoff frequency. This procedure is illustrated in Figure 3b . Taking the experimental difference spectrum of Δ σ 1 ( ω ) with ΔSW ( ω 0 )=0 (blue circle) and carrying out the KK transformation results in the deviation of the real part of the dielectric function from the measured data (blue line in the inset of Fig. 3b ). Only by increasing the SW below ω 0 =12 meV to 0.015 eV 2 (red circle) does one achieve complete agreement with the experiment (red line in the inset). The exact shape of the extrapolated Δ σ 1 ( ω ) has a minor role. The maximum uncertainty introduced by the unknown shape can be calculated as the difference of two extreme configurations: all ΔSW ( ω 0 ) at ω =0 and ω = ω 0 : when ω ≫ ω 0 . On the other hand, the accuracy with which the SW is determined at the same energy is given by The relative effect of the shape change over the magnitude change in the SW in the extrapolation region is then for ω ≫ ω 0 . In the present case taking ω 0 =12 meV and ω =250 meV (as in the inset of Fig. 3b ), one obtains a shape uncertainty of 0.2%. Thus, the effect is negligible already at rather low frequencies. The same analysis applies for the high-energy extrapolation above 6.5 eV. However, complete agreement between Δ ɛ 1 ( ω ) and Δ ɛ 2 ( ω ) within the accuracy of the experiment was found up to 6.5 eV, therefore, no experimentally discernible missing SW is present at higher energies. How to cite this article: Charnukha, A. et al . Superconductivity-induced optical anomaly in an iron arsenide. Nat. Commun. 2:219 doi: 10.1038/ncomms1223 (2011).